Skyrmion flow near room temperature in an ultralow current density The manipulation of spin textures with electric currents is an important challenge in the field of spintronics. Many attempts have been made to electrically drive magnetic domain walls in ferromagnets, yet the necessary current density remains quite high (~10 7 A cm −2 ). A recent neutron study combining Hall effect measurements has shown that an ultralow current density of J ~10 2 A cm −2 can trigger the rotational and translational motion of the skyrmion lattice in MnSi, a helimagnet, within a narrow temperature range. Raising the temperature range in which skyrmions are stable and reducing the current required to drive them are therefore desirable objectives. Here we demonstrate near-room-temperature motion of skyrmions driven by electrical currents in a microdevice composed of the helimagnet FeGe, by using in - situ Lorentz transmission electron microscopy. The rotational and translational motions of skyrmion crystal begin under critical current densities far below 100 A cm −2 . Magnetization dynamics under electric current excitation, such as magnetic domain wall (MDW) motion, has an essential role in spintronic devices. Extensive experimental [1] , [2] , [3] and theoretical [4] , [5] studies have shown that a current on the order of 10 5 –10 8 A cm −2 is capable of moving the conventional MDW or magnetic vortex in ferromagnetic (FM) nanostructures. However, such high current densities should induce the intense joule heating, which is detrimental for practical applications. Among the versatile magnetic nanostructures that could be used as electrically controllable information carriers, the skyrmion (that is, the nanometric vortex-like spin-swirling object) is attracting significant interest as one of the important candidates. The drive of the skyrmion by electric current excitation was first evidenced by a recent neutron scattering study [6] ; an ultralow electric current density on the order of 10 2 A cm −2 can rotate (and hence possibly slide) the skyrmion crystal through the spin-transfer torque and the Magnus force, which was realized in a helimagnet MnSi at lower temperatures (26–28 K). Compared with the conventional case of current-driven MDW motion, much lower power consumption enables one to manipulate skyrmions, which is a promising characteristic for magnetic memory elements in spintronics. Skyrmions arise most typically from helical spin structures induced by the Dzyaloshinskii-Moriya (DM) interaction [7] , [8] in chiral-lattice magnets. Recent experimental observations [9] , [10] , [11] , [12] have confirmed the theoretical prediction [13] , [14] , [15] that skyrmions in a helimagnet are made up of downward (upward) core (peripheral) spins and inside swirling spins; the unique spin-swirling direction of a skyrmion is determined by the underlying crystal symmetry (chirality) governing the sign of the DM interaction. A skyrmion carrying a topological quantum number acts as an internal magnetic flux on the moving electrons. As the electron traverses the skyrmion, it should gain a quantum Berry phase and senses the effective Lorentz force induced by its scalar spin chirality, giving rise to the topological Hall effect [16] . When the electric current, flowing on the skyrmion texture, exceeds a critical density for depinning, the curved spin texture in the skyrmion can accept the spin transfer torque, as in the case of the current-induced MDW motion [17] , to be driven along the current direction [6] . Indeed, the spin-motive force (emergent electric field) due to the translational skyrmion crystal motion has been detected as the correction of the Hall voltage for MnSi [18] . On the other hand, as a counteraction of the above topological Hall effect, the skyrmion or skyrmion crystal itself can exhibit a Hall motion in the direction transverse to the flowing current. Compared with the skyrmion phase forming temperatures (26–28 K) for MnSi, the FeGe thin film shows the formation of a skyrmion crystal in a much wider temperature region (up to 275 K) [12] . Their nanometric magnetic configurations and their spin textures, as directly observed by Lorentz transmission electron microscopy (TEM) [12] , are presented in Fig. 1 . In this study, we target a helimagnetic FeGe thin plate and investigate the skyrmion dynamics in exciting electric currents and in magnetic fields applied normal to the thin plate plane in terms of the real-space and real-time observation with Lorentz TEM. It was observed that skyrmion flow occurs above the critical electric current of less than 10 2 A cm −2 , that is, several orders of magnitude smaller than the critical current for driving MDW motion in FM nanostructures. 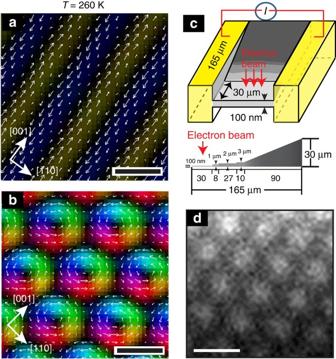Figure 1: Lorentz TEM images and diagram of a microdevice for the observation of current-driven skyrmion motion. (a,b) The in-plane magnetization textures of the helical structure (B=0) and of the skyrmion crystal (B=150 mT), as deduced from the transport-of-intensity equation analysis of the under-focus and over-focus Lorentz TEM images on a 30-nm-thick FeGe plate. Scale bar, 70 nm. Colours and white arrows are signs of the magnitude and orientation of in-plane magnetizations, whereas the dark colour depicts the upward (downward) spins in the periphery (core) of the skyrmions. (c) Schematic diagram and cross-sectional view of a microdevice with a trapezoidal FeGe plate that is composed of a 100 nm-thick thinner terrace for electron-beam transmission and another trapezoidal thicker part for supporting the thinner part. (d) The under-focus Lorentz TEM image for the skyrmion crystal taken at 250 K and 150 mT for the present device. Scale bar (d), 100 nm. Figure 1: Lorentz TEM images and diagram of a microdevice for the observation of current-driven skyrmion motion. ( a,b ) The in-plane magnetization textures of the helical structure ( B =0) and of the skyrmion crystal ( B =150 mT), as deduced from the transport-of-intensity equation analysis of the under-focus and over-focus Lorentz TEM images on a 30-nm-thick FeGe plate. Scale bar, 70 nm. Colours and white arrows are signs of the magnitude and orientation of in-plane magnetizations, whereas the dark colour depicts the upward (downward) spins in the periphery (core) of the skyrmions. ( c ) Schematic diagram and cross-sectional view of a microdevice with a trapezoidal FeGe plate that is composed of a 100 nm-thick thinner terrace for electron-beam transmission and another trapezoidal thicker part for supporting the thinner part. ( d ) The under-focus Lorentz TEM image for the skyrmion crystal taken at 250 K and 150 mT for the present device. Scale bar ( d ), 100 nm. Full size image Spin textures in a microdevice Figure 1a,b present the results of the transport-of-intensity equation analysis of the Lorentz TEM images for proper-screw spin textures under zero magnetic field and skyrmion crystal under 150 mT in a 30-nm-thick FeGe plate at 260 K, respectively [12] . The magnitude and orientation of the in-plane magnetization are represented by the colours and white arrows, while the dark region indicates the magnetization directed along the normal direction. The image taken at zero field in Fig. 1a shows the variation of the in-plane magnetization normal to the helix propagation along [110], indicating a helical period of 70 nm. As a magnetic field is applied normal to the thin plate, the transformation from stripes to the vortex-like skyrmions ( Fig. 1b ) takes place. The dark contrast at outer periphery and the centre of the skyrmions suggests that the peripheral and core spins are parallel and antiparallel to the applied field, respectively. The lattice parameter of the skyrmion crystal (the distance ( d s k ) between adjacent skyrmions) is nearly identical with the period of the helical stripes. We note the formation of a hexagonal skyrmion crystal composed of skyrmions with anticlockwise rotating spins, reflecting the sign of the DM interaction in the single-chiral domain of (110) FeGe. The effect of the dynamic generation and disappearance of the skyrmion crystal on increasing the magnetic field strength was successfully recorded as an in - situ Lorentz TEM image movie (see Supplementary Movie 1 ). The movie unravelled the critical sample thickness dependence of skyrmion formation and its stability; the transformation from helical structure to skyrmion crystal starts from the thinner area (sample edge region) and expands to the thicker area, whereas the disappearance of skyrmions starts from thicker areas (far from the sample edges) with a further increasing field. This result indicates that a thin film can stabilize skyrmions and skyrmion crystals more efficiently. Interestingly, the dynamic rotation of skyrmion crystals while maintaining the chirality has been observed as a changing external field strength, as discerned by a Lorentz TEM movie ( Supplementary Movie 1 ). Translational motion of skyrmions under electric currents Keeping such an active skyrmion motion with a varying normal magnetic field in mind, let us now discuss its manipulation by an electric current. We fabricated the microdevice shown in Fig. 1c , which is composed of a thin small area of FeGe (20 μm×30 μm×100 nm in size) for TEM observations, a thicker supporting part with trapezoid-like FeGe (a schematic and scanning electron microscopy images of FeGe in the device are shown in the lower panel of Fig. 1c and in Supplementary Fig. S1 , respectively), and electronic conducting FeGe blocks on both sides of the thin plates. First, we achieved a Lorentz TEM observation of the thinner part in a zero field. We confirmed the formation of the helical stripes also in this device as the alternating bright/dark regions in the Lorentz TEM image ( Fig. 2a ). Then, we applied a perpendicular magnetic field of 150 mT to create the skyrmion crystal ( Fig. 2e ). The crystal imperfections, such as grain boundaries, are indicated by dashed lines. The fringes of the skyrmion lattice are clearly visualized and extend through the grain boundaries, rendering identical crystal chirality in these grains. Figure 1d shows a magnified image of the skyrmion crystal in region B in this device. Compared with the Lorentz TEM image used in demonstrating the skyrmion crystal spin texture in Fig. 1b , the present image intensity shown in Fig. 1d for this microdevice is weak owing to the increased film thickness (100 nm) that is close to the limit for the electron beam transmittance at an accelerating voltage of 300 kV, but it was nevertheless strong enough to identify the presence of the skyrmion crystal. 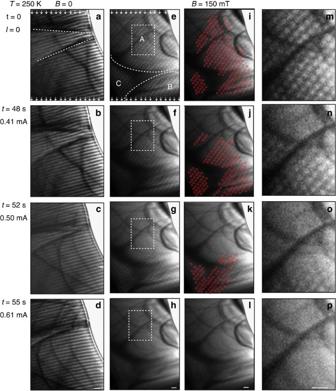Figure 2: Changes in stripes and skyrmions under dc current excitation at 250 K. Lorentz TEM images of variations of the spontaneous helical stripes (a–d) and the skyrmion crystal (e–h) with various currents. A, B and C in (e) are defined as the specific area of the device. (i–l) In the same data shown in (e–h), the skyrmion positions are marked by red circles for clarity. Dashed lines indicate boundaries of crystal imperfections. The white arrows in (a) and (e) indicate the current direction. (m–p) Magnified images of box area A of (e–h). Random dark bent lines in Lorentz configurations indicate the bend contours (equal-inclination fringes). Bright dots represent skyrmions. The current of 1 mA corresponds approximately to the current density 65 A cm−2. Scale bar, 100 nm. Figure 2: Changes in stripes and skyrmions under dc current excitation at 250 K. Lorentz TEM images of variations of the spontaneous helical stripes ( a – d ) and the skyrmion crystal ( e – h ) with various currents. A, B and C in ( e ) are defined as the specific area of the device. ( i–l ) In the same data shown in ( e–h ), the skyrmion positions are marked by red circles for clarity. Dashed lines indicate boundaries of crystal imperfections. The white arrows in ( a ) and ( e ) indicate the current direction. ( m – p ) Magnified images of box area A of ( e – h ). Random dark bent lines in Lorentz configurations indicate the bend contours (equal-inclination fringes). Bright dots represent skyrmions. The current of 1 mA corresponds approximately to the current density 65 A cm −2 . Scale bar, 100 nm. Full size image Next, we show snapshots extracted from Supplementary Movies 2 and 3, which were recorded by Lorentz TEM observations as electric currents were passed through the device. The exposure time and the frame rate are 250 ms and 20 fpm (frames per minute). The current, which was passed from the top-to-bottom direction in these frames, was gradually increased, as indicated in the left part of Fig. 2 . In this device, a current of 1 mA corresponds a current density of ~65 A cm −2 . The irregular shape of the device fabricated by a focussed-ion-beam instrument should affect the accuracy of the current density estimation, but it should not change the order of the current density; the error bar of the absolute magnitude may be at the most ±10%, judging from the irregularity of the plate shape probed by SEM (shown in Supplementary Fig. S1 ). As the current traverses the device at zero magnetic field, essentially no change occurs for the spontaneous helical stripes; the snapshots shown in Fig. 2a–d and Supplementary Movie 2 indicate that the stripes representing the proper-screw magnetic structure remain nearly intact while the electric current is increased. This lack of change also ensures that the joule heating in the observing device induced by such a low current (<0.7 mA) should not increase the device temperature up to the magnetic transition temperature (~275 K). The minimal heating effect on the magnetic contrast should be maintained on the same sample area under identical current excitation conditions even when a static magnetic field as small as 150 mT is applied to generate the skyrmion crystal. We note that the helical stripes structure is robust under current excitation of this magnitude. In Fig. 2e–h , we show the Lorentz TEM images of nearly the same region under an identical current scan but at B =150 mT applied normal to the device film plane. We marked the skyrmion positions on the same images ( Figs 2i–k ) by red open circles to clearly display the overall motion of the skyrmion crystal. Fig. 2m–p represent magnified views for the white-dashed-line box area in region A. These skymion images and their magnified equivalents ( Fig. 2e–p) clearly show that some skyrmion crystal regions eventually disappear as the current I increase above 0.4 mA, or current density J ~26 A cm −2 . Finally, above I= 0.61 mA or J ~39 A cm −2 , no skyrmion crystal (nor helical) texture is discerned in any region, in contrast to the robust subsistence of the stripes at identical current excitations ( Fig. 2d ). We can interpret the disappearance of the skyrmion crystal pattern as representing the current-driven continuous flow of skyrmions on the basis of the following observations and considerations; the exposure time to take one frame is long enough (250 ms) that the movement of the skyrmion, which in the sliding regime should be much faster than the velocity value (280 nm s −1 ) of the skyrmion crystal lattice constant (70 nm) divided by the exposure time (250 ms), will simply appear as a non-contrast or homogeneously grey image in the Lorentz TEM observation, as typically shown in Fig. 2o–p . According to the spin transfer torque mechanism [5] , the current density of 100 A cm −2 above the critical value can give rise to an MDW velocity on the order of 10 4 nm s −1 , well above the present frame resolution. In a bulk crystal of MnSi, the skyrmion crystal drift velocity ( v d ) was estimated by the aforementioned spin-motive force correction to the Hall effect under current excitation; v d ~10 5 nm s −1 at J ~ J c ~10 2 A cm −2 (ref. 17 ), which is again well above the resolution. Nevertheless, in the course of the fading-out process of the skyrmion crystal image around the critical current flow (for example, 0.4–0.5 mA, shown in Fig. 2j, k ), even the static images of the skyrmion crystal taken at the different time frames are observed to not coincide with each other in either position or the direction of the skyrmion crystal, indicating the occurrence of intermittent slides and rotations of the skyrmion crystal. The thermal melting of the skyrmion crystal induced by joule heating is hardly plausible because the stripe images from the screw spin structure (with a nearly identical transition temperature to the paramagnetic state) appears to be robust under the same current excitation condition but at zero applied field. Another possibility would be the current-induced transformation of the skyrmion crystal to the paramagnetic state or the FM state. However, if the paramagnetic or FM state was stabilized via a type of phase transition by the current flow, it would also be realized on the current excitation on the screw state. On the other hand, weak magnetic fields (<1 mT) generated by the extremely weak currents (<0.7 mA) should be small to fully magnetize a FeGe thin plate of this type (see the magnetic phase diagram in Fig. 4a ). With these considerations on the change of skyrmion crystal images and contrasts, it is concluded from a comparison of the images shown in Fig. 2i–l that the skyrmion or skyrmion crystal exhibits the sliding motion above some critical current that seems to strongly depend on the sample position, or perhaps equivalently on the strength or density of pinning sites; skyrmions start to move from region A at the applied current of 0.41 mA, while they begin to move at a current of 0.50 mA in region B. As the current further increases up to 0.61 mA, skyrmions no longer appear to be static over the whole region. The skyrmion crystal motion may be amenable to such a low-current flow compared with the robust case of the screw states ( Figs 2a–d ) or the conventional domain walls because of the difference in the pinning potentials depending on the topological nature of the magnetic texture; the quantitative aspect remains to be solved in future studies. Figure 4: Temperature dependence of the critical current densities for skyrmion motion. 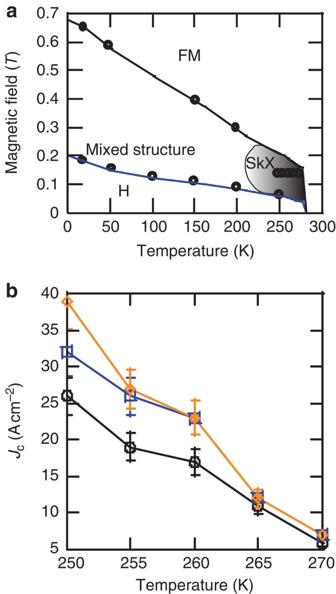Figure 4: Temperature dependence of the critical current densities for skyrmion motion. (a) The schematic phase diagram of the skyrmion crystal in the temperature vs magnetic-field plane. H and FM represent the helical and field-induced spin collinear (FM) state, respectively. Black circles indicate the experimental points, and curved lines show the phase boundaries between H, the mixed state, and the FM state. (b) The temperature dependence of the critical current densityJcfor the skyrmion crystal flow in the FeGe thin plate (100 nm-thick) of the present device at a magnetic field of 150 mT. The orange, blue and black lines represent the data for the different areas shown inFig. 2. The error bars of current density are estimated by the irregularity of the device shape shown inSupplementary Fig. S1. ( a ) The schematic phase diagram of the skyrmion crystal in the temperature vs magnetic-field plane. H and FM represent the helical and field-induced spin collinear (FM) state, respectively. Black circles indicate the experimental points, and curved lines show the phase boundaries between H, the mixed state, and the FM state. ( b ) The temperature dependence of the critical current density J c for the skyrmion crystal flow in the FeGe thin plate (100 nm-thick) of the present device at a magnetic field of 150 mT. The orange, blue and black lines represent the data for the different areas shown in Fig. 2 . The error bars of current density are estimated by the irregularity of the device shape shown in Supplementary Fig. 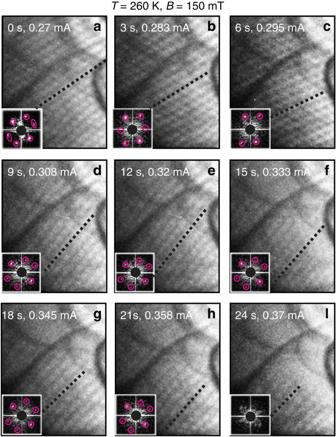S1 . Figure 3: Rotational and translational motions of the skyrmion crystal under current excitation at 260 K. Lorentz TEM images of variations of the skyrmion crystal in a slowly increasing current, as indicated by the elapsed time and current values. Dashed lines represent the orientation of one edge of the skyrmion lattice. The insets show the fast-Fourier-transform patterns of the observation area; the circles in the fast-Fourier-transform patterns represent the positions of the skyrmion lattice, which show random rotations when going from (a) to (e). Translational motion may also occur during the skyrmion crystal rotation. When increasing the current above 0.33 mA, continuous translational motion of the skyrmion crystal appears to occur, as shown in panels (f) to (l). Full size image Rotational motion of skyrmions In addition to the translational motion, the rotational motion of the skyrmion crystal is also discerned in the present device by finely varying the current immediately below the critical value for the sliding motion at 260 K. Figure 3 represents a series of snapshots of Lorentz TEM images with a gradually increasing current (flowing from top to bottom in the figure) around the critical region of the skyrmion flow. The skyrmion crystal dramatically changes its lattice orientation, even before the continuous translational motion. When the current is smaller than 0.27 mA, no change in the skyrmion crystal image appears. As the current increases to 0.28 mA, as shown in Fig. 3b–e , the lattice fringe changes its direction among the respective frames (a dashed line indicates one side of the triangular skyrmion lattice on each frame). This change can also be clearly observed in the fast-Fourier-transform mapping images shown in the respective insets. It is not clear at the moment (but is plausible) that intermittent translational motion may also occur during the skyrmion crystal rotation. For further increases in the current over 0.33 mA, continuous translational motion of the skyrmion crystal appears to occur, extinguishing the skyrmion crystal image ( Fig. 3f–l ). Figure 3: Rotational and translational motions of the skyrmion crystal under current excitation at 260 K. Lorentz TEM images of variations of the skyrmion crystal in a slowly increasing current, as indicated by the elapsed time and current values. Dashed lines represent the orientation of one edge of the skyrmion lattice. The insets show the fast-Fourier-transform patterns of the observation area; the circles in the fast-Fourier-transform patterns represent the positions of the skyrmion lattice, which show random rotations when going from ( a ) to ( e ). Translational motion may also occur during the skyrmion crystal rotation. When increasing the current above 0.33 mA, continuous translational motion of the skyrmion crystal appears to occur, as shown in panels ( f ) to ( l ). Full size image Temperature dependence of J c Thermal agitation is another important factor that affects the skyrmion motion and the skyrmion crystal stability. To verify this effect, detailed investigations were conducted by varying the temperature from 250 K to 270 K in a constant normal-magnetic field of 150 mT. We marked the experimental conditions with open circles in the temperature ( T )-magnetic field ( B ) plane ( Fig. 4a ). On the basis of the Lorentz TEM observation, a crude skyrmion crystal phase diagram is given in Fig. 4a , indicating the presence of a stable skyrmion crystal in a relatively wide ( T , B ) window. In comparison with our previous study [12] , the skyrmion crystal phase in this device seems to be stabilized in the relatively higher magnetic fields, perhaps because the demagnetization effect in such a microdevice may be different from that of the homogeneous thin film with a comparable sample thickness. Figure 4b demonstrates the temperature variation of the critical current J c for driving skyrmions measured at different regions of the view area shown in Fig. 2 . The observed J c is somewhat scattered, depending on the region. On the other hand, it is observed as a generic feature that J c decreases with an increase of the temperature and assumes a smaller value as the skyrmion crystal approaches the paramagnetic transition temperature (~275 K). This tendency is, however, in contradictory with the observation of J c from the change in the Hall effect in a bulk single crystal of MnSi [6] , [18] . This contradiction may be caused by the difference of the pinning effect between two-dimensional skyrmion crystals in the thin film and three-dimensional skyrmion crystals in the bulk. In the case of the pinning due to the local potential minimum, the thermal agitation usually enhances the fluctuation of the particle-like object (skyrmion) and reduces the J c . Therefore, the J c is expected to decrease with temperature as observed in the thin FeGe sample. The present case seems to reflect such an orthodox behaviour, whereas the opposite temperature dependence of the critical current, as observed in the bulk case of MnSi, has been ascribed to the thermal disorder of the three-dimensional skyrmion lattice [6] , [18] . There are several motive forces having key roles in driving skyrmions or skyrmion crystals; the spin transfer torque [6] , the skyrmion Hall effect [19] , and some rotational force acting on the skyrmion crystal. All of these motive forces, as detailed in the following discussions, are in competition with the pinning potential possibly arising from impurities, lattice imperfections, and grain/crystal boundaries. Among them, the spin transfer torque is a well-known mechanism for the current drive of FM MDWs. In the present case, the transfer of spin angular momentum via the spin-polarized current gives rise to torque on the skyrmion spin texture and drags it. As we have observed, the J c for the skyrmion crystal flow is several orders of magnitudes smaller than that for the conventional spin transfer torque mechanism. From the snapshots of the Lorenz TEM pictures alone, we cannot resolve the individual motion of skyrmions; nevertheless, from the pictures of different areas ( Fig. 2 ) and the momentarily still picture ( Fig. 3 ) in the immediate vicinity of J c Hall motion transverse to the current direction as well as the rotational motion of the whole skyrmion crystal is convincingly anticipated to occur in the actual device. As already mentioned, the Hall motion of the skyrmion itself can be anticipated as the counteraction to the topological Hall effect of the spin-polarized current [19] . As for the rotational motion, the former neutron diffraction of bulk MnSi under current excitation was able to successfully capture the phenomena with a comparably low current density (~100 A cm −2 ) [6] . In that case, the origin of the rotation was successfully accounted for in terms of the macroscopic temperature gradient along the current flow, causing the combination of drag and Magnus forces. In the present case, however, the thermal gradient over the small and thin (~100 nm) view area is less plausible, and hence we seek another mechanism; this behaviour might be ascribed to the spin–orbit interaction mediating the coupling between the skyrmion crystal and the underlying chemical lattice, as theoretically proposed recently [20] , or to the deformation of the skyrmion crystal lattice affected by the sample boundaries/dislocations. The origin of the behaviour remains elusive at the moment. In conclusion, real-space and real-time observations were performed near room temperature on the current-driven motion of skyrmions in a microdevice composed of a FeGe thin plate. It was found that a dc current much less than 100 A cm −2 was capable of inducing translational and rotational motion of a skyrmion crystal. The minimum critical current density for moving skyrmions seemed to be as small as 10 A cm −2 , which is several orders of magnitude smaller than the magnitude of the current density (~10 7 A cm −2 ) for controlling domain wall motion in the FM nanostructures. J c for the skyrmion drive was observed to increase with a decrease in the temperature. Skyrmion-based devices with such low-current controllability could be a target of research for next-generation spintronics. Microdevice preparation Our real-time and real-space observations were carried out using a microdevice made up of a trapezoidal FeGe thin plate and two electrical conducting blocks on two sides of the thin plate. The device was fabricated by a focussed-ion-beam instrument (Hitachi FB-2100) equipped with a gallium ion gun. The trapezoidal-shaped FeGe was composed of two parts, which were fabricated as a 100-nm-thick thinner part for electron-beam transmittance and another trapezoidal thicker part for supporting the thinner part. The electrical conducting blocks were made of FeGe-bulk-coated with an Au-Pd layer. The dc current was supplied by a source-measure instrument (KEITHLEY 2611A). Assuming that the current density flowing in the trapezoidal FeGe thin plate was uniform, the current I= 1 mA in this device corresponded approximately to a current density of 65 A cm −2 . Lorentz TEM and transport-of-intensity equation method Lorentz TEM is a power tool for the real-space demonstration of nanometric magnetic domains. The analyses of Lorentz TEM images with the transport-of-intensity equation provide a quantitative magnetic component mapping image. The principle for Lorentz TEM observation is described below. When the electron beam travels through a magnetic material, the Lorentz force induced by the in-plane magnetic components should deflect the beam, resulting in converging (bright contrast) or diverging (dark contrast) on the defocussed (under- or over-focussed) image planes. The inversion of such magnetic contrast can be observed between the under- and over-focussed images [21] . To perform quantitative in-plane magnetizations in Lorentz TEM configurations we analysed the Lorentz TEM images by using a software package QPt [22] , which is based on the transport-of-intensity equation [23] , I ( xyz ) and φ ( xyz ) represent the intensity and electron phase, respectively. On the other hand, Maxwell-Ampére equations lead to a relationship between φ ( xyz ) and the magnetization of the magnetic material as where t is the sample thickness and is the unit vector perpendicular to the sample surface. We can obtain the in-plane magnetization distribution M xy, as φ ( xyz ) is known. φ ( xyz ) can be obtained by equation (1) if ∂ I /∂ z is known. The differential electron intensity around the focussed plane (∂ I /∂ z )(z~0) can be estimated with an approximation where Δz is the defocussed distance and f 1 ( ≫ Δz) is the focal length of the objective lens. This approximation means that the lateral magnetizations can be obtained by analysing the variations of electron intensity in a series of defocussed Lorentz TEM images. How to cite this article: Yu, X.Z. et al . Skyrmion flow near room temperature in an ultralow current density. Nat. Commun. 3:988 doi: 10.1038/ncomms1990 (2012).